A gustatory receptor involved in host plant recognition for oviposition of a swallowtail butterfly Swallowtail butterflies belonging to the family of Papilionidae selectively utilize a limited number of plants from a single or a few families. Female butterflies lay eggs on their host only when they detect specific chemicals through their foreleg chemosensilla while drumming on the leaf surface. Here we show that the butterfly, Papilio xuthus , uses a gustatory receptor specific for synephrine to select its host in oviposition behaviour. We identify a gustatory receptor gene involved in the recognition of an oviposition stimulant, synephrine, from the P. xuthus by a combination of in silico , in vitro and in vivo approaches. The receptor, PxutGr1, responds specifically to synephrine in Sf9 cells. The sensitivity of tarsal taste sensilla to synephrine and the oviposition behaviour in response to synephrine are strongly reduced after injecting double-stranded RNA of PxutGr1 into pupae. These observations indicate that the receptor PxutGr1 represents a key factor in host specialization in P. xuthus . Host selection behaviour is thought to be a key process involved in diversification of phytophagous (plant-feeding) insects. Many lepidopteran species have evolved to select a limited range of host plants, the most extreme state being monophagous feeding on a single species. Swallowtail butterflies, which belong to the family of Papilionidae , selectively utilize a limited number of plants belonging to a single or a few families. A correlation is observed between changes in host plants and diversification of species of this butterfly family [1] . Because host selection arises from oviposition behaviour of female butterflies, oviposition preference is a key determinant of the association between phytophagous insects and their host plants. Butterflies drum on the surface of leaves to ascertain host plant identity before laying eggs [2] , [3] . Using artificial leaves soaked with extracts or specific compounds prepared from host plant leaves, chemicals referred to oviposition regulators, stimulants or repellents, have been identified [4] , [5] . A number of oviposition regulating compounds have been identified for swallowtail butterfly species in the genus Papilio , most members of which feed exclusively on the two plant families, Rutaceae and Apiaceae [6] , [7] , [8] . Extensive analysis by Nishida's group has identified ten oviposition stimulants in Papilio xuthus [9] . Foreleg tarsi, in particular fifth tarsomeres of female butterflies, contain collections of sensilla. The structure and possible function in oviposition behaviour of the sensilla have been studied in the large white butterfly Pieris brassicae [10] . Each sensillum contains four chemosensory neurons and one mechanosensory neuron. The function of the sensillum neurons of P. brassicae was examined by electrophysiological response of the sensillum to water, salts and an oviposition stimulant suggesting a possible role of the neurons in oviposition behaviour [10] . The similarity to P. brassicae , both in oviposition behaviour and in the structure of sensilla in foreleg fifth tarsomeres, suggests that sensilla of P. xuthus foreleg tarsi are also responsible for recognition of oviposition stimulants. Furthermore, we supposed that receptors similar to the gustatory receptors of Drosophila melanogaster are located in sensillum neurons and have a key role in recognition of stimulants and subsequent signal transduction that leads to induction of oviposition behaviour. To date, however, there has been no study on the molecular mechanisms underlying the function of chemosensory neurons in oviposition behaviour, primarily because of the difficulty in identifying receptor genes functioning in insect chemosensory neurons. An important breakthrough was achieved by the whole genome sequencing of D. melanogaster , which revealed a group of 60 genes predicted to encode 68 7-transmembrane proteins (7TMP) as gustatory receptors (Gr) together with 62 7TMPs as olfactory receptors (Or) through in silico and gene expression analyses [11] , [12] , [13] , [14] , [15] , [16] . Among the 60 Gr genes, Gr5a has been identified as a receptor specific for trehalose through genetic and biochemical approaches [17] , Gr5a and Gr64a function as heterodimeric receptors with other members of the Gr family in vivo [18] , Gr66a is expressed in caffeine-sensitive neurons [19] and Gr21a and Gr63a together mediate CO 2 detection [20] . Another Gr gene ( Gr68a ), which may be involved in courtship behaviour of male Drosophila , functions in pheromone reception [21] . The complete genome sequence of Anopheles gambiae , Apis mellifera and Bombyx mori has revealed Gr and Or gene families [22] , [23] , [24] , [25] homologous to those in Drosophila . Using this information on insect gustatory receptor genes, we initiated a study of oviposition behaviour based on gustatory genes functioning in foreleg tarsal sensilla of butterflies. We chose P. xuthus as a test organism, because its oviposition behaviour and oviposition stimulants have been extensively studied [9] . Additionally, P. xuthus is the most common species of swallowtail and can be raised throughout the year with artificial food. Our strategy was first to identify genes for Grs functioning in tarsal sensilla from a set of expression signature tags (ESTs) expressed in female foreleg fifth tarsomere, second to identify the ligands of the receptors by expressing them in Spodoptera frugiperda 9 (Sf9) cells and using a calcium imaging assay, and finally to analyse receptor gene function in the sensilla and in oviposition behaviour. Conventional genetic methods to analyse gene function in vivo , such as gene mutation or gene knockout, are not available in P. xuthus . Therefore, we established an in vivo method to interfere with receptor gene function by double-stranded RNA (dsRNA), as the methods have been successfully applied for various genes in several insect species [26] , [27] , [28] , [29] . Here we report on the identification of a Gr for synephrine, one of ten oviposition stimulants of P. xuthus , and elucidate its function both in the electrophysiological response of tarsal sensilla to synephrine and in oviposition behaviour of females. 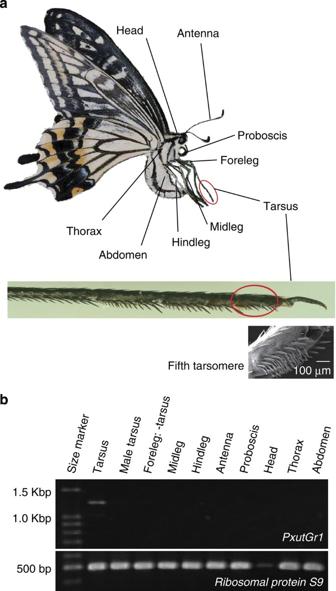Figure 1: A picture ofP. xuthusand organ-specific expression ofPxutGr1. (a) Organs examined for gene expression are indicated with magnification of the fifth tarsomere by SEM. 50–70 sensilla are located on the fifth tarsomere of female forelegs. (b) RT–PCR ofPxutGr1on RNA isolated from various organs. All organs except male tarsi were isolated from single females. RNA extraction and RT–PCR were performed, as described in Methods. Identification of a gustatory receptor gene from P. xuthus The butterfly, P. xuthus and its various organs used in this study are illustrated in Figure 1a . We searched for complementary DNA (cDNA) encoding putative Grs among more than 20,000 ESTs [30] expressed in the female tarsi of P. xuthus by in silico analysis tuned to a 7TMPs characteristic of insect Grs. We first searched for EST sequences containing two or more transmembrane (TM) regions as defined by SOSUI [31] and TMHMM [32] , and subsequently determined the entire sequence of the cDNA clones represented by the ESTs. Using reverse transcription polymerase chain reaction (RT–PCR), we examined whether or not clones were expressed preferentially in female tarsi ( Fig. 1b ). One of the cDNA clones that fit our criteria was 1,224 bp in length and encoded a 407aa open reading frame containing 7TM regions ( Fig. 2a ). To confirm the validity of the cDNA, we cloned the corresponding gene from a P. xuthus genomic library [30] . The gene consists of eight exons encoding the identical 407aa protein ( Supplementary Fig. S1 ). The predicted 7TM protein belongs to the class of insect gustatory receptors as shown by phylogenetic analysis ( Supplementary Fig. S2 ). We found that the gene was indeed expressed preferentially in female tarsi ( Fig. 1b ). We have therefore named the gene as P. xuthus Gr1 ( PxutGr1 ). We were unable to detect the expression of the gene in female tarsi of P. xuthus by either Northern analysis or in situ hybridization, suggesting that expression of the gene is extremely low, similar to the low expression levels seen for D. melanogaster gustatory receptors [13] . Further attempts to identify extra Gr genes from the cDNA library have been unsuccessful, with the possible exception of one 7TM receptor clone, Pxft01604 , similar to the rhodopsin type G protein-coupled receptor of many animal species. However, this gene is expressed ubiquitously and, thus, is unlikely to encode a bona fide Gr. Figure 1: A picture of P. xuthus and organ-specific expression of PxutGr1 . ( a ) Organs examined for gene expression are indicated with magnification of the fifth tarsomere by SEM. 50–70 sensilla are located on the fifth tarsomere of female forelegs. ( b ) RT–PCR of PxutGr1 on RNA isolated from various organs. All organs except male tarsi were isolated from single females. RNA extraction and RT–PCR were performed, as described in Methods. 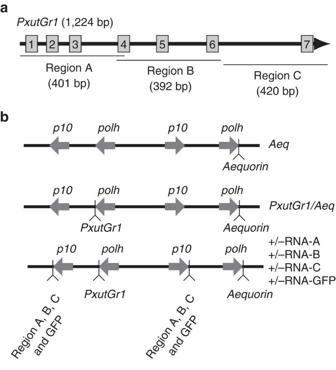Figure 2: Structure of recombinant genes in baculovirus. (a) Structure of coding region ofPxutGr1. Numbered grey boxes represent 7TM regions. Regions A–C are portions of thePxutGr1used for expression of sense and anti-sense RNA and also for preparation of dsRNA. (b) Relative locations of four promoters in the cloning region of baculovirus genome. InAeqvirus, theaequoringene was inserted downstream ofpolhpromoter. InPxutGr1/Aeqvirus,aequorinandPxutGr1genes were inserted downstream of twopolhpromoters in opposite directions. In +/−RNA-A, B, C and GFP viruses, regions A (guanine+cytosine content: 39.4%), B (34.1%), C (37.6%) ofPxutGr1and a 415-bp portion of theGFPgene (34.9%) were inserted downstream of twop10promoters together withPxutGr1andaequoringenes. Full size image Figure 2: Structure of recombinant genes in baculovirus. ( a ) Structure of coding region of PxutGr1 . Numbered grey boxes represent 7TM regions. Regions A–C are portions of the PxutGr1 used for expression of sense and anti-sense RNA and also for preparation of dsRNA. ( b ) Relative locations of four promoters in the cloning region of baculovirus genome. In Aeq virus, the aequorin gene was inserted downstream of polh promoter. In PxutGr1 / Aeq virus, aequorin and PxutGr1 genes were inserted downstream of two polh promoters in opposite directions. In +/−RNA-A, B, C and GFP viruses, regions A (guanine+cytosine content: 39.4%), B (34.1%), C (37.6%) of PxutGr1 and a 415-bp portion of the GFP gene (34.9%) were inserted downstream of two p10 promoters together with PxutGr1 and aequorin genes. Full size image Ligand determination for PxutGr1 by calcium imaging assay Ten compounds have been identified from citrus leaves that stimulate oviposition of P. xuthus [9] . To determine whether any of these ten compounds functions as a ligand for PxutGr1, we performed in vitro assays using the baculovirus expression system. We first prepared a transfer plasmid containing PxutGr1 and Aequorin (Aeq, Ca-dependent luminescence protein) genes ( Fig. 2b ), and introduced them into baculoviruses in Sf9 cells. We confirmed the simultaneous expression of the two genes after 90 h infection of Sf9 cells by the recombinant (PxutGr1/Aeq , Fig. 2b ) virus with multiplicity of infection of 0.5. The exact virus dosage and the period of its propagation were both essential for obtaining consistent results ( Supplementary Fig. S3 ). We examined the effects of candidate compounds on the PxutGr1 receptor expressed in Sf9 cells. A dramatic response of the infected cells was observed when the whole extract of the citrus leaf was used as a stimulant ( Fig. 3a,b ). Using nine of the ten known stimulants for P. xuthus oviposition ( Supplementary Fig. S4 ; vicenin-2 was not commercially available) we observed that only synephrine caused an increase in Ca-dependent luminescence as effectively as the whole citrus extract ( Fig. 3a,b ; Supplementary Fig. S5 ). Sequential stimulation and washing of cells using various stimulants showed that the same cell population responded only to synephrine ( Fig. 3c ). Moreover, the Sf9 cells expressing PxutGr1 did not respond to chemicals closely related in structure with synephrine ( Supplementary Figs S6 and S7 ), with the exception of octopamine. As Sf9 cells have been reported to have an endogenous rhodopsin type G protein-coupled receptor activated by both octopamine and synephrine [33] , we tested Sf9 cells infected with a virus expressing the Aequorin gene alone and found that they responded to synephrine as well as octopamine ( Fig. 3a and b ). However, this endogenous activity for synephrine was much lower than the activity induced by PxutGr1 and it differed significantly in its dependency to the ligand concentration ( Fig. 3d ). It should be noted that the endogenous activity for octopamine was not affected by introduction of PxutGr1 ( Fig. 3a and b ). Furthermore, treatment of PxutGr1 -expressing cells with mianserin, an antagonist of neural octopamine receptor [34] , [35] , [36] , completely inhibited the response to octopamine without affecting the response to synephrine ( Fig. 3e,f ). The response to synephrine was not affected by various concentration of mianserin indicating that there was no competitive interaction between mianserin and synephrine ( Fig. 3f ). In contrast, mianserin showed competitive inhibition on the response to octopamine and synephrine by the endogenous receptor with a similar kinetics ( Fig. 3f ). These results strongly suggest that PxutGr1 encodes a gustatory synephrine receptor that is different from the endogenous octopamine receptor. 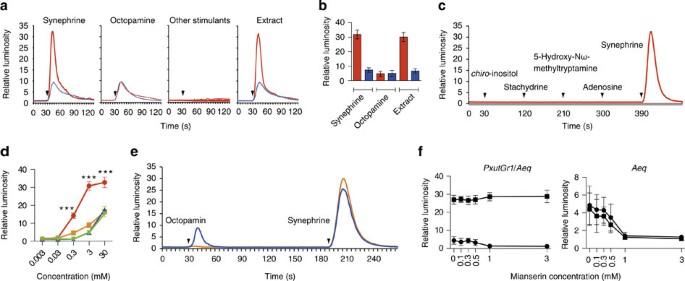Figure 3: Ca-dependent response to oviposition stimulants in Sf9 cells expressingPxutGr1andaequoringenes. (a) Relative luminosity elicited by various compounds. 0.2 ml test solution (30 mM) was pulsed for 2 s to a Petri dish containing 2 ml cell culture at the time indicated by arrowhead (PxutGr1/Aeqcells: red lines,Aeqcells: blue lines). Relative luminosity indicates folds increase in luminosity produced by a given chemical over the luminosity value immediately before the addition of the compound normalized to 1. Stimulants are shown above each figure. Other stimulants are listed inSupplementary Figures S4, S5, S6 and S7. (b) Relative luminosity was measured as in (a). Bars represent mean value (N=8–10) and error bars show standard deviation (s.d.). (c) Five stimulants (30 mM) were added sequentially to the samePxutGr1/Aeqcells in a single Petri dish as shown. (d) Relative luminosity was measured as in (a) using various concentrations of synephrine and octopamine added toPxutGr1/Aeqcells andAeqcells (red: Synephrine toPxutGr1/Aeq; blue: Octopamine toPxutGr1/Aeq; orange: Synephrine toAeq; green: Octopamine toAeq). The mean values (N=5) were plotted against each concentration of added solutions (concentration in cell culture was∼1/10 of each value). Error bars represent s.d. Asterisks indicate the statistical significance between the synephrine inPxutGr1/Aeqcells andAeq(0.3 mM:P=0.00007; 3 mM:P=0.00007; 30 mM:P=0.00007; two-way ANOVA with Tukey HSD). (e) Octopamine and synephrine (30 mM each, final concentration in cell culture was∼3 mM) were sequentially pulsed toPxutGr1/Aeqcells with (orange) or without (blue) mianserin in a Petri dish at times indicated. In experiments with mianserin, cells were maintained in Ringer's solution containing 3 mM mianserin throughout. (f) Relative luminosity was measured as in (e).PxutGr1/AeqandAeqcell cultures containing various concentration of mianserin were sequentially pulsed with 30 mM of synephrine (square) and octopamine (circle). Plots represent mean value (N=6–10) and error bars show s.d. Figure 3: Ca-dependent response to oviposition stimulants in Sf9 cells expressing PxutGr1 and aequorin genes. ( a ) Relative luminosity elicited by various compounds. 0.2 ml test solution (30 mM) was pulsed for 2 s to a Petri dish containing 2 ml cell culture at the time indicated by arrowhead ( PxutGr1 / Aeq cells: red lines, Aeq cells: blue lines). Relative luminosity indicates folds increase in luminosity produced by a given chemical over the luminosity value immediately before the addition of the compound normalized to 1. Stimulants are shown above each figure. Other stimulants are listed in Supplementary Figures S4, S5, S6 and S7 . ( b ) Relative luminosity was measured as in ( a ). Bars represent mean value ( N =8–10) and error bars show standard deviation (s.d.). ( c ) Five stimulants (30 mM) were added sequentially to the same PxutGr1/Aeq cells in a single Petri dish as shown. ( d ) Relative luminosity was measured as in ( a ) using various concentrations of synephrine and octopamine added to PxutGr1 / Aeq cells and Aeq cells (red: Synephrine to PxutGr1 / Aeq ; blue: Octopamine to PxutGr1 / Aeq ; orange: Synephrine to Aeq ; green: Octopamine to Aeq ). The mean values ( N =5) were plotted against each concentration of added solutions (concentration in cell culture was ∼ 1/10 of each value). Error bars represent s.d. Asterisks indicate the statistical significance between the synephrine in PxutGr1 / Aeq cells and Aeq (0.3 mM: P =0.00007; 3 mM: P =0.00007; 30 mM: P =0.00007; two-way ANOVA with Tukey HSD). ( e ) Octopamine and synephrine (30 mM each, final concentration in cell culture was ∼ 3 mM) were sequentially pulsed to PxutGr1 / Aeq cells with (orange) or without (blue) mianserin in a Petri dish at times indicated. In experiments with mianserin, cells were maintained in Ringer's solution containing 3 mM mianserin throughout. ( f ) Relative luminosity was measured as in ( e ). PxutGr1/Aeq and Aeq cell cultures containing various concentration of mianserin were sequentially pulsed with 30 mM of synephrine (square) and octopamine (circle). Plots represent mean value ( N =6–10) and error bars show s.d. Full size image Inhibition of PxutGr1 expression in Sf9 cells by dsRNA To further discriminate the PxutGr1 receptor-dependent activity from that of the endogenous receptor in Sf9 cells, we examined the effect of dsRNA targeted to three regions of PxutGr1 ( Fig. 2a ). We constructed viruses containing each of the three regions of PxutGr1 A, B or C, in both orientations together with PxutGr1/Aeq genes, such that the two strands of RNA (+/−RNA), and hence dsRNA, would be produced simultaneously with the expression of PxutGr1 in the infected Sf9 cells ( Fig. 2b ). As expected, the expression of PxutGr1 became undetectable by RT–PCR for each of the three PxutGr1/Aeq /+/−RNA (A, B or C) constructs. In contrast, similar amount of expression of both genes were observed in control ( Fig. 4a ). We confirmed that the nucleotide sequences of the PxutGr1 exons in these constructs remained intact for each of the expression experiments. Cells infected with PxutGr1/Aeq /+/−RNA virus indeed showed a response to synephrine that was decreased to the endogenous levels seen in Aeq virus-infected control cells ( Fig. 4b and c ). The effect of +/−RNA was specific for the PxutGr1 because a similar construct containing +/−RNA derived from the green fluorescent protein ( GFP ) gene had no effects ( Fig. 4b,c ). These results confirmed that the high-level response to synephrine by the Sf9 cells infected with PxutGr1/Aeq virus was caused by the expression of PxutGr1 and the low-level response observed in the Aeq virus-infected cells was caused by the endogenous octopamine/synephrine receptor in the Sf9 cells. We constructed a baculovirus expressing +/−RNA derived from the endogenous octopamine/synephrine receptor to inhibit its activity in infectious cells. However, we did not observe decrease in the endogenous activity by the +/–RNA. We assume that the endogenous receptor proteins that were formed and integrated within the cell membrane before infection with baculovirus maintained its function even after the expression of dsRNA. 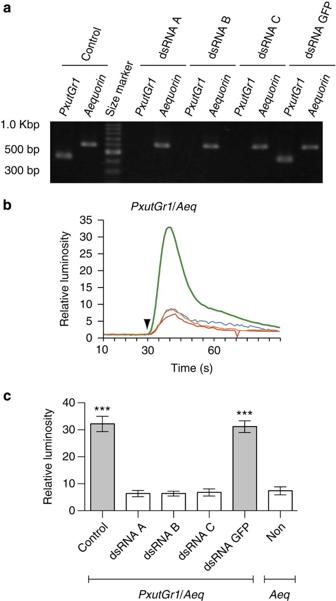Figure 4: Effect ofPxutGr1dsRNAs on the expression and function ofPxutGr1gene in Sf9 cells. (a) Expression ofPxutGr1andaequorinin Sf9 cells infected with baculovirus containing various recombinant genes. Sf9 cells growing in tissue culture flasks were infected with each recombinant baculovirus. Cell extracts were prepared after 90 h and total RNAs were purified. (b) Effect of dsRNAs. Synephrine solution (30 mM) was added at the time indicated by an arrowhead. Green line:PxutGr1/Aeqexpressing cells co-expressed with dsRNA for GFP. The cells expressing dsRNA forPxutGr1are: region A (blue), B (orange) and C (red). (c) Relative luminosity was measured as in (b). Bars show mean value (N=5) and error bars show s.d. Asterisks indicate statistical significance from Aeq virus (PxutGr1/Aeq:P=0.00009996345; dsRNA GFP:P=0.00009996345; one-way ANOVA with Tukey's HSD test). Figure 4: Effect of PxutGr1 dsRNAs on the expression and function of PxutGr1 gene in Sf9 cells. ( a ) Expression of PxutGr1 and aequorin in Sf9 cells infected with baculovirus containing various recombinant genes. Sf9 cells growing in tissue culture flasks were infected with each recombinant baculovirus. Cell extracts were prepared after 90 h and total RNAs were purified. ( b ) Effect of dsRNAs. Synephrine solution (30 mM) was added at the time indicated by an arrowhead. Green line: PxutGr1 / Aeq expressing cells co-expressed with dsRNA for GFP. The cells expressing dsRNA for PxutGr1 are: region A (blue), B (orange) and C (red). ( c ) Relative luminosity was measured as in ( b ). Bars show mean value ( N =5) and error bars show s.d. Asterisks indicate statistical significance from Aeq virus ( PxutGr1 / Aeq : P =0.00009996345; dsRNA GFP: P =0.00009996345; one-way ANOVA with Tukey's HSD test). Full size image Responses of sensilla to synephrine and inhibition by dsRNA We next asked whether PxutGr1 functions in vivo as the receptor for synephrine in the chemosensilla of foreleg tarsi of P. xuthus . We performed electrophysiological recordings [37] using foreleg tarsi freshly cut from adult butterflies within 2 days post eclosion ( Supplementary Fig. S8 ). On the fifth tarsomere of each foreleg, there are ∼ 50–70 sensilla ( Fig. 1a; Supplementary Fig. S8 ). These sensilla are multiply innervated and can be divided into two types, long (L) and short (S), based on their size. Given that the type L sensilla show higher specificity for oviposition stimulants, we examined ∼ 20 L-type sensilla chosen at random from a single tarsomere, as their number and positions varied among individuals. Almost every sensillum examined responded to citrus extracts, as well as to a number of stimulants such as synephrine, stachydrine and chiro -inositol ( Fig. 5a ; Supplementary Fig. S9 ), although size and frequency of spikes were variable among various stimulants ( Supplementary Fig. S9 ). Two criteria were used to estimate the strength of the responses. One was the percentage of sensilla that responded to a given stimulus; the other was the frequency of spikes in each responded sensillum. Both criteria were dependent on the concentration of stimulants and, therefore, were used as quantitative measurement of the electrophysiological responses ( Fig. 5 ; Supplementary Fig. S9 ). 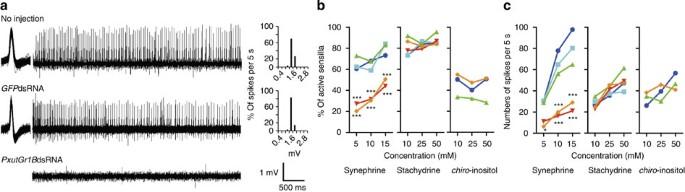Figure 5: Responses of sensilla on the fifth tarsomere of normal and RNAi butterflies to oviposition stimulants. (a) Typical electrophysiological recordings in response to 25 mM synephrine for 5 s obtained from a single sensillum of female individuals as in Methods. Left and right figure of traces show spike sorting and histogram with their amplitudes. No injection was used as control.GFPdsRNA: dsRNA of GFP was injected.PxutGr1BdsRNA:PxutGr1dsRNA region B was injected. (b) Percentage of sensilla that responded to stimulants shown at the bottom of the figure (dark-blue circle: no injection; light-blue square: water injection; green triangle:GFPdsRNA injection; red inverted triangle:PxutGr1AdsRNA injection; orange diamond:PxutGr1BdsRNA injection). Activities of approximately 20 sensilla were measured from normal and 10 μg dsRNA injected (RNAi) individuals 5 days before eclosion. Asterisks indicate statistical significance fromGFPdsRNA injection (Region A 5 mM:P=7.508E-07; 10 mM:P=0.00008; 25 mM:P=0.000027; Region B 5 mM:P=6.463E-08; 10 mM:P=0.000098; 25 mM:P=0.000543, two-way ANOVA with Fisher LSD). (c) Frequency of spikes was measured from 5 s recordings. Colors and symbols are the same as in (b). Asterisks indicate statistical significance fromGFPdsRNA injection (Region A 5 mM:P=0.0324; 10 mM:P=0.00003; 25 mM:P=9.0547E-07; Region B 5 mM:P=0.0065; 10 mM:P=0.00001; 25 mM:P=0.0000117; two-way ANOVA with Fisher LSD). Figure 5: Responses of sensilla on the fifth tarsomere of normal and RNAi butterflies to oviposition stimulants. ( a ) Typical electrophysiological recordings in response to 25 mM synephrine for 5 s obtained from a single sensillum of female individuals as in Methods. Left and right figure of traces show spike sorting and histogram with their amplitudes. No injection was used as control. GFP dsRNA: dsRNA of GFP was injected. PxutGr1B dsRNA: PxutGr1 dsRNA region B was injected. ( b ) Percentage of sensilla that responded to stimulants shown at the bottom of the figure (dark-blue circle: no injection; light-blue square: water injection; green triangle: GFP dsRNA injection; red inverted triangle: PxutGr1A dsRNA injection; orange diamond: PxutGr1B dsRNA injection). Activities of approximately 20 sensilla were measured from normal and 10 μg dsRNA injected (RNAi) individuals 5 days before eclosion. Asterisks indicate statistical significance from GFP dsRNA injection (Region A 5 mM: P =7.508E-07; 10 mM: P =0.00008; 25 mM: P =0.000027; Region B 5 mM: P =6.463E-08; 10 mM: P =0.000098; 25 mM: P =0.000543, two-way ANOVA with Fisher LSD). ( c ) Frequency of spikes was measured from 5 s recordings. Colors and symbols are the same as in ( b ). Asterisks indicate statistical significance from GFP dsRNA injection (Region A 5 mM: P =0.0324; 10 mM: P =0.00003; 25 mM: P =9.0547E-07; Region B 5 mM: P =0.0065; 10 mM: P =0.00001; 25 mM: P =0.0000117; two-way ANOVA with Fisher LSD). Full size image To demonstrate that PxutGr1 is responsible for the response to synephrine in tarsal sensilla, we prepared adult female butterflies injected with PxutGr1 dsRNA to inhibit expression of PxutGr1 in tarsal sensilla. As controls, we injected either water or dsRNA prepared from a portion of GFP gene similar in size and guanine+cytosine content with PxutGr1 dsRNA. In all cases, survival rates due to injection were more than 95%. We first confirmed by quantitative RT–PCR that expression of PxutGr1 was indeed inhibited in the tarsi when the PxutGr1 dsRNA was injected into pupae more than 3 days before eclosion ( Fig. 6 ). We next examined the responses of tarsal taste sensilla from butterflies injected with PxutGr1 dsRNA: we name them as interference RNA (RNAi) butterflies ( Fig. 5a ). In the RNAi butterflies, the response to synephrine, but not to stachydrine and chiro -inositol was strongly inhibited both in the percentage of responded sensilla ( Fig. 5b ) and in the number of spikes elicited in these responding sensilla ( Fig. 5c ; Supplementary Fig. S9a ). We observed the reduction in the responses to synephrine specifically by dsRNA from both regions A and B of PxutGr1 when injected 5 days before eclosion. In contrast, control injections of water and GFP dsRNA had no effects. These results argue that PxutGr1 encodes a synephrine receptor that functions in taste sensilla of foreleg tarsi. 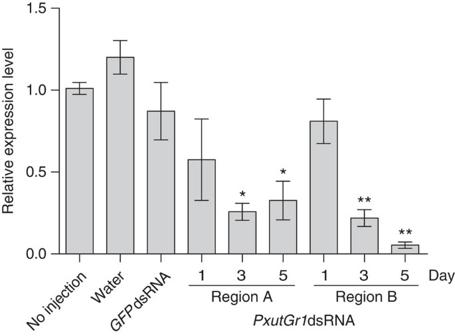Figure 6: Expression of thePxutGr1in dsRNA-injected butterflies and controls. In all cases, total RNA was extracted from foreleg tarsi of each individual butterfly within 2 days after eclosion. One μg of RNA was used for quantitative RT–PCR using specific primers forPxutGr1andribosomal protein S17. Amounts of PCR product relative to that of no injected individuals are shown with variations of 2–6 individuals. Water andGFPdsRNA were injected 5 days before eclosion.PxutGr1dsRNA region A or B was injected 1, 3, or 5 days before eclosion, as indicated in abscissa. Asterisks indicate statistical significance fromGFPdsRNA injection (Region A, 3 days:P=0.00075; Region A, 5 days:P=0.00207; Region B, 3 days:P=0.00042; Region B, 5 days:P=0.00018; one-way ANOVA with Fisher LSD). Figure 6: Expression of the PxutGr1 in dsRNA-injected butterflies and controls. In all cases, total RNA was extracted from foreleg tarsi of each individual butterfly within 2 days after eclosion. One μg of RNA was used for quantitative RT–PCR using specific primers for PxutGr1 and ribosomal protein S17 . Amounts of PCR product relative to that of no injected individuals are shown with variations of 2–6 individuals. Water and GFP dsRNA were injected 5 days before eclosion. PxutGr1 dsRNA region A or B was injected 1, 3, or 5 days before eclosion, as indicated in abscissa. Asterisks indicate statistical significance from GFP dsRNA injection (Region A, 3 days: P =0.00075; Region A, 5 days: P =0.00207; Region B, 3 days: P =0.00042; Region B, 5 days: P =0.00018; one-way ANOVA with Fisher LSD). Full size image Effect of dsRNA on oviposition behaviour of butterflies Finally, we tested the effects of dsRNA on the oviposition behaviour of female adult butterflies. Re-examination of oviposition stimulants for P. xuthus under carefully controlled conditions confirmed previous reports [9] that the combination of two compounds, synephrine and chiro -inositol, could replace the mixture of ten known stimulants or the citrus whole extract with an efficiency of ∼ 72%. In contrast, either synephrine or chiro -inositol alone failed to stimulate oviposition ( Table 1 ). Encouraged by this finding, we examined the effects of dsRNA for the PxutGr1 B region on the induction of oviposition behaviour stimulated by synephrine and chiro -inositol. The PxutGr1B dsRNA was injected into female pupae 5 days before eclosion, and the oviposition behaviour of RNAi butterflies was examined 3–5 days post eclosion. As controls, we injected either water or GFP dsRNA into pupae. As shown in Table 1 , only 21% of RNAi butterflies laid eggs on the artificial leaves, whereas 78% of water-injected and 62% of GFP dsRNA-injected butterflies succeeded in oviposition ( Supplementary Movie 1 ). Drumming behaviour of the RNAi individuals was as active as in the control butterflies, indicating that contact of sensilla with the substrate was similar to controls ( Supplementary Movie 2 ). RNAi butterflies alone showed a prolonged drumming behaviour when they touch their forelegs to artificial leaves applied with the syneprhrine and chiro -inositol mixture. On the other hand, they, like normal individuals, flew away immediately from artificial leaves applied with water or single-compound solutions and laid eggs to artificial leaves applied with the citrus extracts within a few seconds. These results show that deficiency of the PxutGr1 receptor due to dsRNA injection suppressed the oviposition behaviour despite normal physical contact of sensilla with synephrine. In contrast to its effect on the response to artificial leaves treated with synephrine and chiro -inositol, PxutGr1 dsRNA treatment had no effect on the oviposition response to whole citrus extract. This argues that PxutGr1 normally functions in concert with other receptors to other stimulants and that there is redundancy in the ability of these receptors to elicit the oviposition response. In fact, a mixture of 6 stimulants excluding synephrine is capable of eliciting oviposition behaviour [9] . Table 1 The effect of PxutGr1B dsRNA on oviposition behaviour. Full size table We have identified a single Gr gene ( PxutGr1 ) from ∼ 20,000 ESTs (2,116 species) expressed in female foreleg tarsomeres of P. xuthus . Assuming that the butterfly recognizes at least 10 oviposition stimulants, each by a specific Gr in taste cells located in sensilla of tarsomere, we would expect there to be a number of other Gr genes in addition to PxutGr1 . Our failure to isolate further Gr genes from the ESTs is probably because of extremely low expression levels of Gr genes in taste cells, similar to what has been reported for Grs in Drosophila [13] . RT–PCR revealed clearly that PxutGr1 is expressed specifically in the tarsomere of female forelegs. Further attempts to localize the expression by in situ hybridization of sensillum preparations have been unsuccessful, again probably because of low expression of the gene. However, as discussed below, interference of PxutGr1 expression in the tarsomere by PxutGr1 dsRNA (detected by quantitative PCR; Fig. 6 ) paralleled the inhibition of the response of sensilla to the ligand of the PxutGr1 receptor. Collectively, these results indicate that PxutGr1 is expressed in sensilla of the tarsomere. We expressed PxutGr1 in Sf9 cells with the baculovirus infection system. We found that careful control of virus dosages and growth of Sf9 cells, before and after the infection of the recombinant virus, was essential to obtain constant satisfactory results ( Supplementary Fig. S3 ). Among nine oviposition stimulants for P. xuthus , synephrine alone elicited a PxutGr1-dependent Ca response. This response to synephrine could reproducibly be elicited after repeated treatment of the infected cells with compounds that failed to elicit the response. Sf9 cells contain an endogenous receptor for octopamine that is also activated by synephrine [33] , and hence resulted in a background response to synephrine. We overcame this problem by two means. First, we showed that mianserin, an antagonist of the endogenous octopamine/synephrine receptor, effectively eliminated the background response without affecting the PxutGr1 -dependent response. Second, we interfered with PxutGr1 gene expression in Sf9 by dsRNA. As the dsRNA prepared from three portions of PxutGr1 gene added to the Sf9 cell culture did not interfere with the gene expression, we constructed a virus vector containing a portion of the gene in opposite orientations, such that dsRNA was produced simultaneously with the expression of PxutGr1 . As expected, the construct inhibited PxutGr1 expression and consequently eliminated PxutGr1 -dependent response to synephrine without affecting the background response to synephrine and octopamine. Taken together, our results indicate that synephrine specifically induces a change of Ca concentration via signal transduction mediated by the expression of PxutGr1 in Sf9 cells. Receptors for sweet and bitter tastes in Drosophila are known to form heterodimers with co-receptors to recognize the tastant [18] , [19] , [38] , [39] . At the moment, we do not exclude a possibility that PxutGr1 requires a similar co-receptor that may enhance the specific response of the receptor to synephrine in our calcium imaging assay. We examined the expression and function of a Drosophila Gr, Gr5a, in our calcium imaging assay system and found that the receptor responded to its ligand, trehalose, with activity of ∼ 20% of that observed with the PxutGr1-synephrine response. The low activity of Drosophila Gr5a in Sf9 cells may be owing to the fact that the evolutionary distance between Drosophila and Spodoptera is much longer than that between Papilio and Spodoptera . Encouraged by the effective interference of PxutGr1 expression in Sf9 cells by dsRNA, we tested PxutGr1 function in vivo by injecting PxutGr1 dsRNA into pupae at a stage just before the onset of PxutGr1 gene expression. We found that the timing of injection is essential to inhibit PxutGr1 expression in the tarsomeres of females that were ready for oviposition a few days after eclosion ( Supplementary Fig. S10 ). Injection of PxutGr1 dsRNA markedly inhibited electrophysiological responses of tarsi sensillum neurons to synephrine, whereas responses to other stimulants, such as stachydrine and chiro -inositol, were not affected. This suggests that PxutGr1 functions as a synephrine-specific receptor and not as a nonspecific co-receptor such as Orco in the Drosophila olfactory system [40] . Effects of PxutGr1 dsRNA were equally dramatic on the oviposition behaviour of female butterflies elicited by artificial leaves coated with synephrine and chiro -inositol. Oviposition behaviour can be divided into two separate stages: flying, landing and drumming on the leave surface, followed by bending the tail for laying eggs. PxutGr1 dsRNA injection specifically inhibited the second stage without affecting the first (mediated by visual and olfactory cues), indicating that the PxutGr1 receptor functions in the recognition of the stimulant synephrine that leads to the second and last stage of the oviposition behaviour. Usually, normal butterflies quit the drumming behaviour in less than 2 s on artificial leaves either before laying eggs or flying away depending on solutions applied to leaves. RNAi butterflies showed a prolonged drumming on the artificial leaf applied with the mixture of synephrine and chiro -inositol irrespective of whether they lay eggs or fly away after the drumming. In contrast, RNAi butterflies quit the drumming on leaves applied with the other solutions without synephrine as quickly as normal individuals. In addition, RNAi butterflies lay eggs on artificial leaves with the citrus extract after a normal short drumming. We assume that the unusual drumming behaviour of RNAi butterflies was due to incomplete inhibition of the receptor synthesis by RNAi unlike gene knockout. RNAi butterflies try hard (taking a prolonged time) to recognize synephrine using the remaining small amount of receptors either to fail or succeed in oviposition. Interestingly, PxutGr1 dsRNA injection does not affect the oviposition response to whole citrus extract, which contains multiple oviposition stimulants. This suggests that gustatory receptor neurons (GRNs) expressing PxutGr1 function in concert with GRNs for the other stimulants, and that there is redundancy in the capacity of these GRNs to elicit the oviposition response. Our electrophysiological data further confirm that there is some degree of functional redundancy among GRNs in eliciting oviposition behaviour. Such redundancy could underlie a broader tuning of host plant selection beyond a single plant species, thus allowing for flexibility in host plant choice. For example, although P. xuthus has a preferred plant species for oviposition ( Citrus unshiu ), it could retain the ability to recognize and select a number of different plant species, each producing a distinct but overlapping set of chemical cues. Our findings open the way to identifying other receptors for each oviposition stimulant to study the molecular mechanism of signal transduction in these specialized taste receptors and to gain a better understanding of the evolution of host plant selection of the butterfly. Identification of 7TM protein genes from cDNA library A cDNA library was prepared as reported previously [30] . Base calling from chromatograph files was performed with the Phred program [41] . Low-quality bases (quality score <20) were trimmed from both ends of sequences and those shorter than 200 base pairs were removed using the TRIM3 program supplied in the PCAP package [42] . Vector and primer sequences were trimmed using Cross_match supplied in the Phrap package (P. Green, unpublished). High-quality ESTs having more than 200 base pairs were used for assembling by the CAP3 program [43] referring to a file of quality values generated by the phd2fasta program. The assembled DNA sequences were annotated by homology search, using the BLASTX program. Sequences that were not annotated ('no hits found' or 'hit to unnamed genes') were translated into amino-acid sequences by the GENETYX program (Genetyx Corporation). Amino-acid sequence data longer than 60 residues were examined for 7TM protein candidates by the QFC program [44] and annotated by homology search using the BLASTP program. Full-length cDNA sequences of candidate clones were determined by the primer walking method. Amino-acid sequences of coding regions deduced from cDNA were used to analyse the presence or absence of transmembrane regions by the SOSUI [31] or TMHMM [32] algorithm. Reverse transcriptional PCR of PxutGr1 Total. RNA was prepared from each tissue using a QuickGene RNA tissue kit SII (Fujifilm) following the manufacturer's protocols, and treated with DNase I (Takara Bio). Two μg of RNA were used for the first-strand cDNA synthesis by SuperScript II reverse transcriptase (Invitrogen) and 9-mer random primers (Takara Bio). The reaction mixture was diluted tenfold in TE buffer and used for a PCR template. Primers for the entire PxutGr1 and portion of Ribosomal protein S9 are listed in Supplementary Table S1 . The PCR reaction was performed 30 cycles at 95 °C for 30 s, 60 °C for15 s. and 72 °C for 90 s. Construction of a dendrogram of insect cheomoreceptors Amino-acid sequences of insect chemoreceptors [16] , [45] (more detail in Supplementary Fig. S2 legend) available in public databases were aligned using the ClustalW [46] algorithm. The dendrogram was constructed by the maximum likelihood method using RAxML [47] software. Amino-acid sequences of three rhodopsins of Drosophila were used as out-groups (not shown). Construction of recombinant baculovirus PxutGr1 gene and its various portions were amplified by PCR using primers listed in Supplementary Table S1 and inserted downstream of promoters in pBAC 4x-1 Transfer Plasmid (Novagen). Plasmid constructs were transformed into Escherichia coli DH5a Electro-Cells (Takara Bio), using an E. coli pulser (Bio-Rad). Individual transformants were picked and grown overnight in MMI medium (1.3% Bacto trypton, 2.5% Bacto yeast extract, 145 mM NaCl, 0.4% glycerol, 20 mM Tris–Hcl pH7.2), and plasmid DNA was isolated and purified using a QuickGene Plasmid Kit (Fujifilm). Purified plasmids were used to construct recombinant baculoviruses by a flashBAC system (Oxford Expression Technologies) following the manufacturer's instructions. Calcium imaging assay We developed a novel calcium imaging method for insect Grs in Sf9 cells based on the method used by Torfs et al . [48] Sf9 cells were grown in SF-900 II SFM medium (Invitrogen) and infected with recombinant baculoviruses with multiplicity of infection of 0.5. After growing in tissue culture flask for 90 h, cells were transferred to 35 mm Petri dishes and added with Coelenterazine solution. After incubation of the cell culture for 1 h, medium was replaced by 2 ml Ringer's solution (12.5 mM NaCl, 0.5 mM KCl, 0.2 mM CaCl, 0.1 mM MgSO 4 , 1 mM glucose, and 1 mM HEPES) and placed in a detector C8801 (Hamamatsu Photonics, with modifications) for a continuous recording of the low-level luminescent and luminosity by Ca 2+ -activated aequorin. A perfusion system was constructed by modifying the detector to be able to measure luminescent in real-time ( Supplementary Fig. S11a ). Two metal pipes were installed in a tray of the detector and plastic tubes were passed through the pipes ( Supplementary Fig. S11b ). Tubes were connected to a peristaltic pump and vessels were installed with a three-way cock. All compounds were dissolved in Ringer's solution. Test solutions were applied for 2 s using a peristaltic pump driven system (100 μl s −1 .) into Petri dish containing 2 ml of cell culture in Ringer's solution by switching the three-way cock. Test solutions were then washed by Ringer's solution flowing after each stimulation ( Supplementary Movie 3 ). Since the solution flowed continuously at 100 μl s −1 . the concentration of test compounds reached a maximum value within 2 s after application and quickly decreased. The maximum concentration of the cell culture is 1/10 of that of the added solution. This system can stimulate infected cells in a single Petri dish using up to 5 compounds by sequentially switching cocks installed in vessels. dsRNA preparation and injection Double-stranded RNA was prepared as follows: first purified PCR products of DNA region A and B ( Fig. 2a ) were prepared using primers including T7 promoter sequence. Primers are listed in Supplementary Table S1 . Using the PCR products as templates, dsRNA was prepared using Megascript T7 kit (Ambion) following manufacturer's protocol. dsRNA was concentrated to 1 μg μl −1 by ethanol precipitation. Ten μl of the concentrated dsRNA was injected into female pupa 5 days before eclosion, using a capillary syringe (Hamilton; Supplementary Fig. S12 ), because the expression of PxutGr1 begins on 3 days and becomes highest on 1 day before eclosion ( Supplementary Fig. S10 ). Quantitative RT–PCR The experimental procedure is as described in RT–PCR except that the PCR reaction was performed using SYBR Premix EX Taq II (Takara Bio) following the manufacturer's protocols. Primers for a portion of PxutGr1 and ribosomal protein S17 are listed in Supplementary Table S1 . Efficiencies of RT–PCR reaction were determined by TaKaRa Thermal Cycler Dice real time system (Takara Bio) following the manufacturer's protocols. Butterflies Female P. xuthus butterflies were collected in Takatsuki, Osaka, Japan. Eggs were collected in a temperature-controlled breeding room. Larvae were reared on artificial diet (Insecta F-II from Nosan and dried leaves of Zanthoxylum ailanthoides , collected from the field) at 24±2 °C (LD 16:8). Adult females were hand-paired within 2 days after eclosion and fed Pocari Sweat (Otsuka Pharmaceutical) daily. Electrophysiological assay Forelegs of individual females were removed from the insect body using fine forceps and fixed on a polystyrene block. A glass capillary electrode, filled with Ringer's solution, was inserted into the leg and connected to ground ( Supplementary Fig. S8 ). The leg was taped to the support to expose sensilla from the ventral side of the fifth tarsomere. Recordings were made from individual sensillum by covering them with a 10-μm diameter glass capillary electrode filled with 1 mM KCl plus a given compound in solution. The electrode was advanced under visual control with a compound stereo microscope until it capped the tip of a sensillum. The electrical signal was amplified by a TastePROBE amplifier DTP-02 (Syntech) and further amplified and filtered by a CyberAmp 320 (10-2800 Hz; Axon Instruments). Data were recorded and stored on a computer with a 16-bit A/D conversion card DT9803 USB A/D (Data Translation) under the control of dbWave custom software [49] . Recordings were analysed using dbWave ( Fig. 5a ; Supplementary Fig. S9 ), to detect and sort spikes according to their amplitude and shape. Preparation of whole extract from Citrus leaves Young leaves of Citrus spp. were extracted with methanol at room temperature for 1 month. The methanol extract was concentrated in vacuum below 50 °C, and an aliquot of the whole concentrate was dissolved in methanol at 1% by weight. Artificial plastic leaves were soaked in the extracts solution, and dried at room temperature. Test artificial leaves were moistened by misting with ultrapure water immediately before the bioassay. Bioassay for oviposition behaviour Before testing, only those individuals that showed positive responses to the foliage of Citrus spp . were chosen to remove butterflies that would never lay eggs even in fresh leaves because of the mating failure or other unknown reasons. Only less than 5% of individuals were removed by this selection. Each gravid female (hand-paired, 3–5 days old) was fed with Pocari Sweat (Otsuka Pharmaceutical) early in the afternoon as oviposition activity is higher in the afternoon, incubated in a plastic cup for 30 min while they remained wing-closed. Four 12 W fluorescent lights (about 2,200 lux) were turned on after they opened their wings and they were subsequently introduced into a bioassay chamber (w 55 cm×d 55 cm×h 55 cm) after they had begun flapping wings for ∼ 10 min. Artificial leaves were soaked in compounds solutions (30 mM each) immediately before presentation to free flying butterflies. The response of an individual was scored as 'success' individuals for either actual egg-laying or an equivalent behaviour [7] , [9] (to put the ovipositor in contact with the artificial leaf; Supplementary Movie 1 ) and as 'failure' for either drumming only ( Supplementary Movie 2 ) or landing to the artificial leaves without contact of the ovipositor. Scanning electron microscopy Tarsi of female butterflies were fixed and dried. Mounted legs were sputter-coated with gold and observed by a JSM-5300 LV scanning electron microscope (JEOL). Accession code: The sequence for PxutGr1 has been deposited in the DNA Data Bank of Japan database under accession number AB260115 . How to cite this article: Ozaki, K. et al . A gustatory receptor involved in host plant recognition for oviposition of a swallowtail butterfly. Nat. Commun. 2:542 doi: 10.1038/ncomms1548 (2011).